Sponge-like molecular cage for purification of fullerenes Since fullerenes are available in macroscopic quantities from fullerene soot, large efforts have been geared toward designing efficient strategies to obtain highly pure fullerenes, which can be subsequently applied in multiple research fields. Here we present a supramolecular nanocage synthesized by metal-directed self-assembly, which encapsulates fullerenes of different sizes. Direct experimental evidence is provided for the 1:1 encapsulation of C 60 , C 70 , C 76 , C 78 and C 84 , and solid state structures for the host–guest adducts with C 60 and C 70 have been obtained using X-ray synchrotron radiation. Furthermore, we design a washing-based strategy to exclusively extract pure C 60 from a solid sample of cage charged with a mixture of fullerenes. These results showcase an attractive methodology to selectively extract C 60 from fullerene mixtures, providing a platform to design tuned cages for selective extraction of higher fullerenes. The solid-phase fullerene encapsulation and liberation represent a twist in host–guest chemistry for molecular nanocage structures. Fullerenes have a wide range of applications, highlighting their extensive use as electroactive materials in solar cells [1] , [2] , [3] , and with continuously appearing new uses in medicine [4] , [5] . Any application, however, is limited in origin by tedious solid–liquid extractions (usually in toluene) and time-expensive chromatographic separations [6] , [7] , [8] , [9] , [10] , [11] , [12] , [13] , [14] , [15] . More recently, the host–guest chemistry of molecular containers has been explored to encapsulate fullerenes [16] . Still selectivity is usually difficult to achieve because fine modulation of the size of molecular cages to accommodate different fullerenes is challenging with the limitations of covalent synthesis [17] . Host platforms containing extended π-systems have been designed because of their affinity towards the sphere-like unsaturated structure of fullerenes. In this line, several covalent or supramolecular approaches pursued include: (a) macrocyclic arene-based receptors [18] , [19] , [20] , [21] , [22] , [23] , [24] , (b) macrocyclic structures containing aromatic heterocycles [25] , [26] , [27] , [28] , (c) π-extended TTF receptors [29] , [30] , [31] , [32] , [33] and (d) macrocyclic or jaw-like structures containing porphyrin moieties [17] , [34] , [35] , [36] , [37] , [38] , [39] , [40] , [41] , [42] , [43] , [44] , [45] . Interestingly, Fujita and co-workers reported the use of the empty channels of a metal–organic framework (MOF) for encapsulating fullerenes upon soaking MOF crystals in fullerene-containing toluene. This work is remarkable because it explores the ability of a solid crystalline structure to absorb fullerenes into its large pores by displacing solvent molecules [46] . On the other hand, focusing the interest on selective recovery of encapsulated fullerenes, several strategies have been applied to release the guest molecules as detailed in Fig. 1 (refs 17 , 28 , 39 , 45 , 47 , 48 , 49 , 50 ). In all reported examples, however, there is the need to expose the host to chemical or physical treatment to release the sequestered guests, which prevent its straightforward reusability either because it is blocked by a high-affinity secondary guest, or because the host cage is disassembled. In the case of Fujita’s crystalline sponge strategy [46] , the retention capability is high and half lives of inclusion complexes are over 15 days, thus release of fullerenes must be achieved by deconstructing MOF crystals by acid treatment. 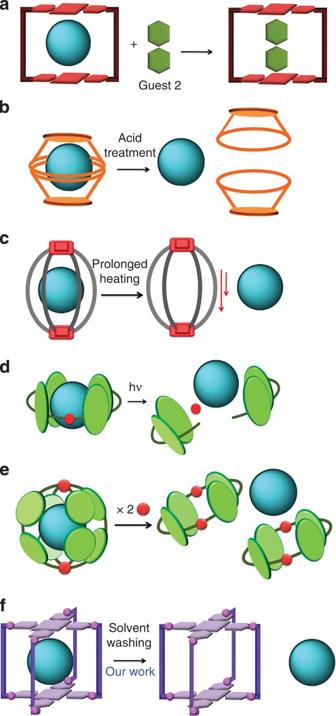Figure 1: Literature precedents for fullerene liberation from fullerene⊂host adducts. (a) Addition of secondary guests in a guest-exchange process17,39,47, (b) acid or base treatment to provoke a structural rearrangement of the host28, (c) prolonged heating to cause the precipitation of the host48, (d) photoreduction of metal ions to disassemble metal-coordination-based supramolecular hosts49, (e) by transforming the shape of the cage in response to an external stimulus50and (f) solid–liquid solvent washing strategy. Figure 1: Literature precedents for fullerene liberation from fullerene ⊂ host adducts. ( a ) Addition of secondary guests in a guest-exchange process [17] , [39] , [47] , ( b ) acid or base treatment to provoke a structural rearrangement of the host [28] , ( c ) prolonged heating to cause the precipitation of the host [48] , ( d ) photoreduction of metal ions to disassemble metal-coordination-based supramolecular hosts [49] , ( e ) by transforming the shape of the cage in response to an external stimulus [50] and ( f ) solid–liquid solvent washing strategy. Full size image Here we present a tetragonal prismatic supramolecular cage with a high affinity for the inclusion of fullerenes and a facile ability to release them by solvent washing of the solid inclusion compound. The cage, built by metal-directed self-assembly of two zinc porphyrin moieties and four molecular clips through Pd coordination bonds, encapsulates exclusively from C 60 to C 84 fullerenes, and C 60 can be selectively released due to their different host affinities. Moreover, the tetragonal prismatic cage design endows four large entrances that enable an unprecedented example of inclusion and release of fullerenes within a molecular cage in the solid state, thus showing a sponge-like behaviour that allows for rapid purification of fullerene mixtures. Synthesis and characterization of 4·(X) 8 cages (X=CF 3 SO 3 or BArF (BArF=tetrakis[3,5-bis(trifluoromethyl)phenyl]borate)) Three-dimensional tetragonal prismatic molecular cage 4 ·(X) 8 was synthesized by self assembly of a tetracarboxylate Zn II -porphyrin and Pd II -based macrocyclic synthons (( Pd-1b )·(AcO) 2 (CF 3 SO 3 ) 2 ). 4 ·(X) 8 differs from the recently described cage 3 ·(X′) 8 (X′=ClO 4 , CF 3 SO 3 ) (ref. 51 ) in the aromatic part of the hexaaza macrocyclic ligands; 3 ·(X′) 8 contained 1,4-substituted benzene rings that have been replaced by biphenyl rings in 1b . As a result, the distance between metalloporphyrins is enlarged from 7.5 Å in 3 ·(X′) 8 to 14.1 Å in 4 ·(X) 8 ( Figs 2 and 3 ). 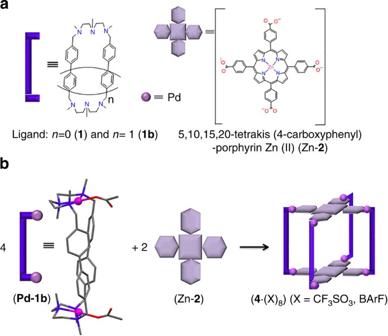Figure 2: Building blocks to obtain the tetragonal prismatic nanocage 4·(X)8. (a) Building blocks used for (b) the self assembly of molecular clipPd-1band tetracarboxylated Zn-porphyrin (Zn-2) to form supramolecular nanocages4·(X)8(X=CF3SO3, BArF), (X-ray diffraction ofPd-1bshows one acetate anion coordinated to each Pd centre, and omits the two triflate counteranions for clarity). Figure 2: Building blocks to obtain the tetragonal prismatic nanocage 4·(X) 8 . ( a ) Building blocks used for ( b ) the self assembly of molecular clip Pd-1b and tetracarboxylated Zn-porphyrin (Zn- 2 ) to form supramolecular nanocages 4 ·(X) 8 (X=CF 3 SO 3 , BArF), (X-ray diffraction of Pd-1b shows one acetate anion coordinated to each Pd centre, and omits the two triflate counteranions for clarity). 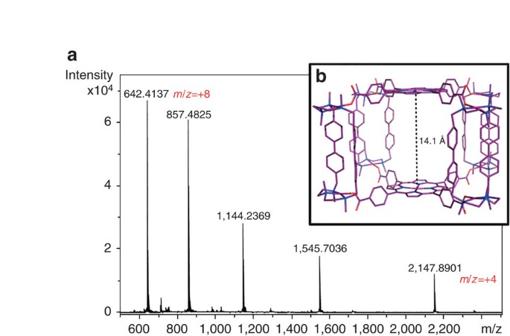Figure 3: Characterization of 4·(BArF)8. (a) HRMS of4·(BArF)8. (b) Representation of48+extracted from X-ray diffraction data. Full size image Figure 3: Characterization of 4·(BArF) 8 . ( a ) HRMS of 4 ·(BArF) 8 . ( b ) Representation of 4 8+ extracted from X-ray diffraction data. Full size image Cage 4 ·(CF 3 SO 3 ) 8 was characterized in solution by electrospray ionization mass spectrometry (ESI-MS). However, the compound was poorly soluble in organic solvents. Improved solubility was exhibited by 4 ·(BArF) 8 , which was isolated in 38% yield after anion exchange. The high resolution mass spectrometry (HRMS) spectrum of 4 ·(BArF) 8 shows ions corresponding to the cage with consecutive loss of counteranions, demonstrating its integrity in solution ( Fig. 3a ). Furthermore, full NMR characterization was performed for 4 ·(BArF) 8 , showing that it has a D 4h symmetric structure in solution. Importantly, the diffusion-ordered spectroscopy nuclear magnetic resonance (DOSY NMR) experiment afforded a diffusion coefficient of D =3.1 × 10 −10 m 2 s −1 , indicating that the dimensions of 4 8+ correspond to a hydrodynamic radius of 19.0 Å in solution, in line with the value estimated from crystallographic data (17.4 Å; see Supplementary Table 1 ). The dimensions of 4 8+ derived from DOSY NMR are, as expected, larger than in tetragonal cage 3 8+ (ref. 51 ). Crystallographic data were obtained from 4 ·(BArF) 8 crystals at the XALOC beamline of the ALBA Synchrotron ( Fig. 3b ) [52] using MD2M single-axis diffractometer (Maatel, France) and a Pilatus 6 M detector (Dectris, Switzerland). Due to its sensitivity to solvent loss, a crystal of 4 ·(BArF) 8 was measured mounted in a thin glass capillary suspended in ether/dimethylformamide (DMF) (solution used to grow the crystal saturated with ether) and cryopreserved at 100 K. The crystal showed poor diffraction data with reflections of moderate intensity which were further degraded rapidly after 266 degrees oscillation (equivalent to 200 s of collection). This poor density and fast degradation (seen in all measured crystals, including both nanocages 4 8+ with encapsulated C 60 and C 70 - vide infra -) could be attributed to the high symmetry, solvent loss and severe motions of the solvents (volatile diethyl ether) and counteranions BArF − molecules in the large cavities of the crystal lattice (see additional comments to X-ray diffraction data in the Supplementary Discussion ). All these reasons hampered a complete X-ray diffraction characterization, as counteranions could not be detected and located. Flash cooling the crystals at 100 K by mounting them in a capillary with cryoprotectants did not provide better crystallographic data. However, the correct structural solution for the cationic molecular cage 4 8+ was achieved. As expected, nanocage 4 8+ consists of two parallel tetracarboxylated Zn II -porphyrins (distance between Zn II centres at the porphyrin moieties=14.1 Å) linked by four macrocyclic dinuclear Pd II complexes. The four-carboxylate residues of each porphyrin are linked by means of η 1 -O monodentate coordination to one Pd II centre. Altogether, the overall structure is defined as a tetragonal prismatic cage taking the set of eight equivalent atoms of the carboxyphenyl moieties as vertices of the polyhedron, thus bearing D 4h symmetry. Fullerene encapsulation The large void volume of the cage (approximately able to encapsulate a spherical guest of up to 696 Å 3 ) and the known affinity of zinc-porphyrins for fullerenes [17] , prompted us to explore the capability of 4 ·(BArF) 8 to act as a host for fullerenes. Fast inclusion of C 60 occurred during the mixing of a solution of 4 ·(BArF) 8 in acetonitrile with C 60 in toluene in a 1:1 molar ratio ( Fig. 4 ). Job plot analysis of ultraviolet–visible (UV–vis) titration data indicated the formation of a 1:1 adduct C 60 ⊂ 4 ·(BArF) 8 with a high association constant of K a =2.8 (±0.6)·10 7 M −1 (log K a =7.44±0.1). The association constant was further confirmed by fluorescence titrations (log K a (fluorescence)=7.47±0.03) (see Supplementary Fig. 1 ). In addition, a HRMS of this mixture showed exclusively the peaks corresponding to C 60 ⊂ 4 ·(BArF) 8 . Crystals were grown by diethyl ether diffusion over a toluene/acetonitrile (4/1) solution of C 60 ⊂ 4 ·(BArF) 8 (isolated yield=70%). The 1 H-NMR spectra in CD 3 CN revealed that several aromatic C–H signals had shifted from the spectrum of the empty cage, indicating the inclusion of fullerene in the cage. DOSY NMR experiments afforded a similar hydrodynamic radius for C 60 ⊂ 4 ·(BArF) 8 when compared with that of the empty cage (see Supplementary Table 1 ), demonstrating that the molecular entity had not changed in size upon addition of the fullerene. Crystals of C 60 ⊂ 4 ·(BArF) 8 were also found to be extremely sensitive to solvent loss, therefore we resorted to low temperature X-ray diffraction analysis at the same synchrotron beamline in thin glass capillaries (flash cooling the crystals at 100 K by mounting them in a capillary with cryoprotectants did not afford better diffraction data). As was the case with 4 ·(BArF) 8 , a consistent crystallographic solution of the cationic molecular cage was achieved. The studies showed the presence of a spherical electron density at the centre of the cage that fitted nicely to a disordered entrapped C 60 molecule ( Fig. 4 ). Detection of this C 60 molecule compared with the failure to locate counteranions and solvent guest molecules can be tentatively attributed to its lower mobility inside the cage. Moreover, the computed structure of the host–guest complex C 60 ⊂ 4 ·(Cl) 8 using state-of-the-art DFT methods showed nice agreement with crystallographic data ( Fig. 4 ; all atoms were calculated at density functional theory (DFT) level). DFT calculations indicated that different orientations of C 60 inside the host are accessible (see Supplementary Table 2 ), thus accounting for the disordered fullerene molecule found in the crystallographic structure. 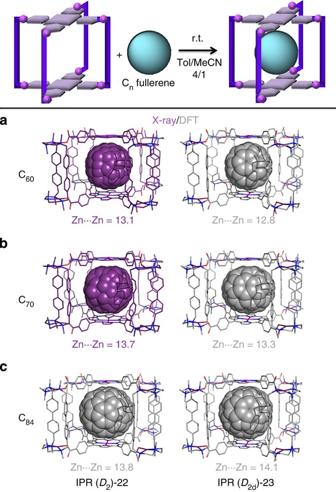Figure 4: X-ray diffraction and DFT analysis of fullerene host–guest compounds. Crystallographic data (purple) and DFT structures (grey) for cationic fullerene inclusion compounds (a) C60⊂48+and (b) C70⊂48+; and (c) DFT calculation for C84⊂48+isomers IPR (D2)-22 and IPR (D2d)-23 (Zn···Zn distances in Å). r.t., room temperature. Figure 4: X-ray diffraction and DFT analysis of fullerene host–guest compounds. Crystallographic data (purple) and DFT structures (grey) for cationic fullerene inclusion compounds ( a ) C 60 ⊂ 4 8+ and ( b ) C 70 ⊂ 4 8+ ; and ( c ) DFT calculation for C 84 ⊂ 4 8+ isomers IPR ( D 2 )-22 and IPR ( D 2d )-23 (Zn···Zn distances in Å). r.t., room temperature. Full size image We then explored the encapsulation of C 70 with 4 ·(BArF) 8 following an equivalent procedure as for C 60 ( Fig. 4 ). C 70 ⊂ 4 ·(BArF) 8 was instantaneously obtained upon mixing host and guest in a 1:1 ratio. UV–vis titration, 1 H-NMR and HRMS showed a very favourable association and stability of the inclusion complex in solution. Due to the high affinity of the cage towards the C 70 , we were unable to obtain an association constant using UV–vis titrations; we therefore resorted to flurorescence titrations and we obtained log K a =8.6±0.3 M −1 (see Supplementary Fig. 2 ), which is roughly 10-fold higher than for C 60 . DOSY NMR spectrum also indicated the same diffusion coefficient as for C 60 ⊂ 4 ·(BArF) 8 and 4 ·(BArF) 8 , thus suggesting that C 70 is also occupying the inner space of the cage with no substantial volume modification of the whole cage. Crystals were grown by diethyl ether diffusion and measured under synchrotron radiation. Similar problems of location of counteranions and rapid loss of crystallinity were encountered, but yet the data collected allowed identifying the structure of the cationic molecular cage including an ellipsoid-shaped electron density at the centre of the cage that fits nicely to a disordered C 70 molecule, finding the semi-major axis parallel to the porphyrin planes ( Fig. 4 ). DFT calculations indeed indicate that this arrangement is ~ 6 kcal·mol −1 more stable than the perpendicular alignment. As observed in the case of C 60 , different orientations of the C 70 molecule with the semi-major axis parallel to the porphyrin planes are accessible, thus indicating that the fullerene moiety can easily rotate (see Supplementary Table 3 ). The DFT-optimized C 70 ⊂ 4 ·(Cl) 8 structure also showed nice agreement with crystallographic data ( Fig. 4 ; all atoms were calculated at DFT level). Comparison of crystallographic data for 4 ·(BArF) 8 , C 60 ⊂ 4 ·(BArF) 8 and C 70 ⊂ 4 ·(BArF) 8 shows that porphyrin–porphyrin interdistance is maximized (14.1 Å) when guest molecule is absent, whereas the inclusion of C 70 compressed this distance down to 13.7 Å and inclusion of C 60 further shrinks it to 13.1 Å ( Table 1 ). DFT-optimized structures are in line with the observed experimental trends. Therefore, the sum of structural and computational information shows an important degree of adaptability or ‘breathing’ of the cage by maximizing the porphyrin–fullerene interaction (see Supplementary Fig. 3 ). Table 1 Structural data. Full size table Given the large void space of the cage 4 ·(BArF) 8 , we explored the limits of encapsulation of higher fullerenes and chemically modified fullerenes. To that end, we selected the larger C 84 and [60]PCBM ([6,6]-phenyl-C 61 -butyric acid methyl ester). Both of them were encapsulated in a 1:1 fashion forming C 84 ⊂ 4 ·(BArF) 8 and [60]PCBM ⊂ 4 ·(BArF) 8 , as indicated by HRMS. The extremely low solubility of C 84 precluded NMR and UV–vis host–guest studies. On the other hand, HRMS for [60]PCBM ⊂ 4 ·(BArF) 8 also indicated a clean 1:1 adduct and did not show desymmetrization of the 1 H-NMR signals, suggesting that the inner space is large enough to allow free rotation of the anisotropic [60]PCBM. Moreover, model C 84 ⊂ 4 ·(Cl) 8 species were optimized at a DFT level, selecting the two most abundant isomers (( D 2 )-22 and ( D 2d )-23 IPR (Isolated-Pentagon-Rule) isomers, see Fig. 4 and Supplementary Figs 4 and 5 ). The computational investigation of C 84 encapsulation inside the host indicated that the porphyrin–porphyrin interdistance is elongated ~ 0.5 Å with respect to C 70 ⊂ 4 ·(Cl) 8 . This value is similar to the porphyrin–porphyrin distance found for the empty nanostructure, indicating that there exists a good fit between C 84 and the cavity of the host cage. 4 ·(BArF) 8 is thus capable of unusually facile encapsulation of C 60 , C 70 , C 84 and [60]PCBM. Relative affinity for the most abundant and accessible C 60 with respect to C 70 was also explored in a HRMS study; one equivalent of 4 ·(BArF) 8 was mixed with one equivalent of C 60 and one equivalent of C 70 in a 4:1 toluene:acetonitrile solvent mixture. HRMS of the resulting solution showed a preferential encapsulation of C 70 with a 9:1 peak intensity ratio for C 70 ⊂ 4 ·(BArF) 8 versus C 60 ⊂ 4 ·(BArF) 8 . On the other hand, when one equivalent of 4 ·(BArF) 8 is combined with 10 equivalents of C 60 and one equivalent of C 70 , two equally intense signals are found for C 60 ⊂ 4 ·(BArF) 8 and C 70 ⊂ 4 ·(BArF) 8 . Finally, a mixture of one equivalent of 4 ·(BArF) 8 with one equivalent of C 60 and nine equivalents of C 70 completely excludes the noticeable encapsulation of C 60 and C 70 ⊂ 4 ·(BArF) 8 is exclusively observed by HRMS. Substoichiometric additions of C 60 and C 70 confirmed the same MS ionization behaviour of free host, host-C 60 and host-C 70 compounds, meaning that the relative intensity of the peaks corresponding to host-C 60 and host-C 70 with the same charge reproduce their relative concentration in solution. An estimation of the affinity to the host for the two fullerenes could then be extracted from this analysis, revealing that C 70 bears a nine-fold higher affinity for 4 ·(BArF) 8 than C 60 , in agreement with the 10-fold difference in association constants found by fluorescence spectroscopy studies. These results are rationalized by a higher degree of π-interactions with C 70 due to its ellipsoid shape (see Supplementary Figs 7–10 ). This is confirmed by DFT calculations, which indicate a more favourable porphyrin–fullerene interaction for C 70 fullerene molecule (see Supplementary Fig. 11 and Supplementary Tables 3 and 4 ). These results are consistent with the X-ray diffraction data in which C 70 ⊂ 4 ·(BArF) 8 presents a less-strained cage conformation, closer to its form as empty cage 4 ·(BArF) 8 , while the more distorted cage in case of C 60 ⊂ 4 ·(BArF) 8 gives a less stable adduct. The inclusion of fullerenes in 4 ·(BArF) 8 is also observed by using fullerene extract (SES Research, C 60 70%, C 70 28%, higher fullerenes 2%). HRMS of the inclusion compounds formed upon mixing 4 ·(BArF) 8 with fullerene extract (1:3 molar ratio, assuming that all fullerenes are C 60 ) in a mixture of toluene/acetonitrile (4/1) exhibited the ion peaks corresponding to C 60 ⊂ 4 ·(BArF) 8 , C 70 ⊂ 4 ·(BArF) 8 and C 84 ⊂ 4 ·(BArF) 8 as the main signals, although minor ion peaks corresponding to C 76 ⊂ 4 ·(BArF) 8 and C 78 ⊂ 4 ·(BArF) 8 were also observed. The C 60 ⊂ 4 /C 70 ⊂ 4 and C 70 ⊂ 4 /C 84 ⊂ 4 ratios derived from the relative intensity of the ion peaks are 0.72 and 12.8, respectively. However, when using different excesses of fullerene, enrichment of the proportion of higher fullerenes caged was observed. Thus, for 1:12 cage:fullerene extract molar ratios, mass spectra affords C 60 ⊂ 4 /C 70 ⊂ 4 and C 70 ⊂ 4 /C 84 ⊂ 4 ratios of 0.18 and 11.3, respectively, whereas larger excess (1:60 weight ratio) afforded C 60 ⊂ 4 /C 70 ⊂ 4 and C 70 ⊂ 4 /C 84 ⊂ 4 ratios of 0.05 and 6.7, respectively (see Supplementary Fig. 12 ). Therefore, the initial 30% content of C 70 and higher fullerenes is remarkably improved to >96% after a single extraction with 4 ·(BArF) 8 . On the other hand, when fullerene soot (Aldrich, C 60 5.3%, C 70 1.54%, higher fullerenes 0.14%, the rest being other forms of carbon) is suspended in toluene and reacted with 4 ·(BArF) 8 (1:12 cage:soot weight ratio; final solvent mixture toluene/acetonitrile 4/1), similar ratios of encapsulation as for fullerene extract were found (see Supplementary Fig. 13 ). The versatility of the cage is further exemplified by the fact that encapsulation of fullerenes can be performed by soaking 4 ·(BArF) 8 as a solid (grain size: 3.1±3.0 μm; median: 2.2 μm; Supplementary Fig. 14 ) [53] in a C 70 -containing toluene solution, thus being the first example of solid-phase fullerene encapsulation for a supramolecular cage (to our knowledge, a single similar precedent using a MOF was reported by Fujita and co-workers) [46] . This observation discards partial cage disassembly during the host–guest event, and agrees with a guest encapsulation occurring by fullerene entrance through the four apertures of the cage; the dimensions of the apertures are large enough to envision the mobility of fullerene molecules through them. Moreover, we could also modify the selectivity toward higher fullerenes, using solid 4 ·(BArF) 8 and fullerene extract dissolved in toluene by changing the fullerene extract ratio used (see Supplementary Figs 15–16 ). These results prompted us to investigate the encapsulation of C 70 dissolved in toluene and insoluble 4 ·(CF 3 SO 3 ) 8 as solvent-evacuated crystals. After 5–10 min, complete inclusion was obtained forming C 70 ⊂ 4 ·(CF 3 SO 3 ) 8 , as ascertained by HRMS ( Supplementary Fig. 17 ). Once the inclusion of fullerenes (from C 60 to C 84 ) was thoroughly studied, we sought to find a straightforward experimental protocol to liberate the different fullerenes in a selective manner. Taking advantage of the fact that fullerenes are encapsulated in the solid state, we charged solid 4 ·(BArF) 8 nanocapsule (0.33 μmols) together with Celite in a short column. Subsequently, a 1.4 mM solution of C 60 was passed through the column seven times, and total encapsulation was confirmed by HRMS. Afterwards, the extraction of C 60 from the solid sample of C 60 ⊂ 4 ·(BArF) 8 charged in the column was performed by consecutive washings with 1,2-dichlorobenzene/CS 2 (1/1 v/v mixture). This solvent mixture fulfills the requirements of a very high solubility of fullerenes and very low solubility of either C 60 ⊂ 4 ·(BArF) 8 or 4 ·(BArF) 8 . We were delighted to observe that washing with 5 × 1 ml of the 1,2-dichlorobenzene/CS 2 mixture was sufficient to liberate all encapsulated C 60 (see Fig. 1f ). On the other hand, the solid remaining in the filtration column was found to be 4 ·(BArF) 8 , which was ready to be filled again with C 60 . The solid fullerene encapsulation–extraction protocol was repeated up to five cycles (see flow chart in Supplementary Fig. 18 ). After these cycles, 91% of 4 ·(BArF) 8 was recovered from the column by washing with acetonitrile ( Fig. 5a ). To the best of our knowledge, this is the first example of the use of orthogonal solubility of the host and fullerene for the extraction of fullerenes (only the reverse adsorption of fullerenes by soaking a MOF crystal in fullerene-containing toluene was reported by Fujita and co-workers) [46] . 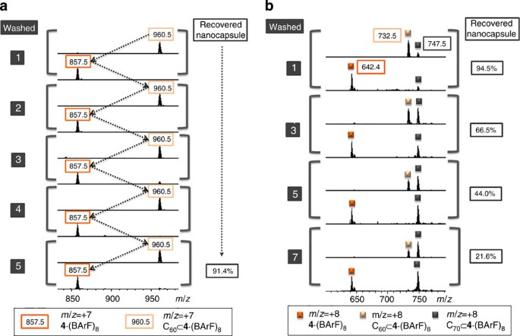Figure 5: Solid state extraction of fullerenes from 4·(BArF)8. HRMS monitoring of the C60extraction washing-protocol using (a) pure C60encapsulated in4·(BArF)8in the solid phase and (b) fullerene extract encapsulated in4·(BArF)8. Figure 5: Solid state extraction of fullerenes from 4·(BArF) 8 . HRMS monitoring of the C 60 extraction washing-protocol using ( a ) pure C 60 encapsulated in 4 ·(BArF) 8 in the solid phase and ( b ) fullerene extract encapsulated in 4 ·(BArF) 8 . Full size image The same protocol was attempted for the inclusion of a mixture of fullerenes (fullerene extract). However, ineffective mixing at the column between the solid 4 ·(BArF) 8 and the toluene solution containing fullerene extract afforded inhomogeneous distribution of fullerenes among the solid. We therefore decided to improve the encapsulation step by re-dissolving the empty cage in CH 3 CN and performing the encapsulation of fullerene extract in solution (1:1 molar ratio). Subsequently, the fullerene-containing cage was precipitated out by the addition of diethyl ether and the filled cage reintroduced in the column (see Supplementary Fig. 19 ). At the first cycle, C 60 ⊂ 4 /C 70 ⊂ 4 ratio was 4.0 (by HRMS), and only C 60 was released after washing the solid inclusion compound with 1,2-dichlorobenzene/CS 2 (1/1 v/v mixture). After repeating the inclusion and liberation sequence up to seven cycles ( Fig. 5b ), the cage was enriched with C 70 at each cycle and was finally saturated of mainly C 70 and C 84 (an ~ 10% mass loss was observed after each cycle due to the experimental setup). The maximum extraction capacity was calculated as 1 mol of C 60 per mol of cage 4 ·(BArF) 8 , and a 61% of the expected C 60 was recovered (quantified by UV–vis). Overall, this experiment demonstrates that the simple and fast selective C 60 purification from a mixture of fullerenes is feasible by using cage 4 ·(BArF) 8 and our solvent-washing protocol [54] . Regarding the recovery of higher fullerenes (mainly C 70 and C 84 ) trapped in the saturated sample of 4 ·(BArF) 8 after multiple encapsulation/liberation cycles, we tested other solvent mixtures but no significant liberation of higher fullerenes was achieved. Therefore, we resorted to triflic acid (10 equivalents) treatment (in toluene) of C 70 and C 84 ⊂ 4 ·(BArF) 8 in the solid state to disassemble the cage and rapid release of the mixture of higher fullerenes into toluene solution. Further partial reassembly of cage 4 ·(CF 3 SO 3 ) 8 upon base (NEt 3 ) neutralization and reflux in DMF occurred, as ascertained by HRMS (see Supplementary Fig. 20 ). To sum up, we have designed the new molecular cage 4 ·(BArF) 8 that encapsulates fullerenes (from C 60 to C 84 ) in a fast manner at room temperature. At the core of the adaptability of the cages to bind substrates that differ substantially in size is the remarkable ability to modulate the size of the cavities by alteration of porphyrin–porphyrin distances. This molecular ‘breathing’ ability of the cages relies on the substantial degree of flexibility of metal-coordination (Pd-carboxylate) bonds in the clips that hold the supramolecular structure. Full spectroscopic and spectrometric characterization of the host and host–guest compounds is reported. In addition, a sponge-like behaviour has been proven for 4 ·(BArF) 8 for the selective purification of C 60 from a mixture of fullerenes. This study provides fundamental results regarding the ability of the described tetragonal nanocage to encapsulate and liberate fullerenes, and paves the way to study the performance of newly designed cages (varying the nature of metalloporphyrin moieties, decorating the apertures of the cage, changing Pd cations at the molecular clips by first-row transition metals, and so on) to finely tune the selectivity for higher fullerenes or endohedral fullerenes. Here we demonstrate for the first time that the encapsulation event can occur by soaking the molecular nanocage in the solid state in a fullerene-containing toluene solution. Moreover, the liberation of C 60 is also achieved by applying solvent-washing protocols to the host–guest complex in the solid state. We envision these findings may spark supramolecular host-guest research in the solid phase in cages bearing apertures for guest entrance. Materials and instrumentation Reagents and solvents used were commercially available reagent quality unless indicated otherwise. Ligand H2pp (see Supplementary Fig. 21 ) was synthesized according to published procedures [55] . NMR data concerning product identity were collected on Bruker 400 MHz AVANCE spectrometers in CDCl 3 or CD 3 CN, and calibrated relative to the residual protons of the solvent. ESI-MS experiments were collected and analysed on both a Bruker Daltonics Esquire 6000 spectrometer and a Bruker MicroTOF-Q-II, using acetonitrile or DMF as the mobile phase. UV–vis spectroscopy was performed on an Agilent 8452 UV–vis spectrophotometer with 1 cm quartz cell, equipped with a temperature control cryostat from Unisoku Scientific Instruments (Japan), using a toluene/acetonitrile 9/1 (v/v) mixture as solvent. Fluorescence measurements were performed in a Spectrofluorimeter Fluorolog Horiba Jobin Yvon. Synthesis and characterization of 1b ligand 0.66 g of H2pp (1.2 mmols) are added to a 100 ml flask and mixed with: 10 ml of formaldehyde, 8 ml of formic acid and 10 ml of water. The resulting mixture is heated to reflux during 12 h. After this time, the reaction mixture is cooled to room temperature and the solvent removed under reduced pressure. Then 25 ml of NaOH 30% are added. The product is extracted with CHCl 3 (3 × 25 ml). Organic phases are combined, dried with anhydrous MgSO 4 and filtered. The remaining solution is dried under vacuum, and the obtained product purified by recrystallization with acetone. (Yield: 51.8%). 1 H-NMR (400 MHz, CDCl 3 ) δ p.p.m. : 7.39 (d, J =8.24 Hz, 8H, arom), 7.29 (d, J =8.24 Hz, 8H, arom), 3.47 (s, 8H, CH 2 ), 2.57–2.49 (m, 16H, CH 2 ), 2.28 (s, 6H, CH 3 ), 2.22 (s, 12H, CH 3 ). 13 C-NMR (75 MHz, CD 3 CN) δ p.p.m. : 139.5 (arom), 137.9 (arom), 129.5 (arom), 126.7 (arom), 62.3 (–CH 2 – benzylic), 54.8 (–CH 2 –), 54.4 (–CH 2 –), 43.6 (N–CH 3 ), 42.9 (N–CH 3 ). Fourier transform infrared (spectroscopy) ν (cm −1 ): 1,462 (C–N st), 1,650–2,000, 2,780 (C–H st, sp 3 ), 2,935 (arC–H st), 2,967 (C–H st, sp 2 ). ESI-MS ( m / z ): calculated 647.9 and found 647.4 ({Me2pp+H} + ). For NMR and ESI-MS analysis of 1b , see Supplementary Figs 21–25 . Synthesis and characterization of 1b·(AcO) 2 (CF 3 SO 3 ) 2 molecular clip In a round-bottom flask, 0.08 g of 1b ligand (0.125 mmols), 0.058 g of Pd(AcO) 2 (0.250 mmols) and 25 ml of anhydrous CH 3 CN were mixed. The mixture is heated to reflux temperature, under nitrogen atmosphere for 18 h. After this time, the reaction mixture is cooled down to room temperature. Subsequently, an excess of NaCF 3 SO 3 salt is added (0.525 mmols) and the mixture is stirred vigorously for 6 h. The reaction mixture is concentrated to a volume of 2–3 ml under reduced pressure, filtered through Celite and recrystallized under slow diethyl ether diffusion. Yellow crystalline solid is obtained. (Yield: 90.1%). 1 H-NMR (400 MHz, CD 3 CN) δ p.p.m. : 8.37 (d, J =8 Hz, 10.5 H, arom), 8.15 (d, J =8 Hz, 8 H, arom), 7.94 (d, J =8 Hz, 2.5 H, arom), 4.06 (d, J =13 Hz, 5.25 H, –CH 2 –), 3.62 (m, 5.26 H, –CH 2 –), 3.33 (s, 11.9 H, N–CH 3 ), 3.31 (s, 3.6 H, N–CH 3 ), 3.25 (m, 5.25 H, –CH 2 -), 3.11 (d, J =13 Hz, 5.17 H, –CH 2 –), 2.38 (d, J =14 Hz, 5.0 H, –CH 2 –), 2.30 (d, 5.2 H, –CH 2 –), 2.07 (s, 5.9 H, AcO), 2.05 (s, 1.8 H, AcO), 1.50 (s, 1.8 H, N–CH 3 ), 1.41 (s, 6.0 H, N–CH 3 ). 13 C-NMR (100 MHz, CD 3 CN) δ p.p.m. : 178.7 (C=O, AcO), 142.2 (arom), 141.03 (arom), 133.8 (arom), 133.6 (arom), 128.5 (arom), 128.1 (arom), 65.6 (–CH 2 –), 65.4 (–CH 2 –), 61.0 (–CH 2 –), 60.8 (–CH 2 –), 59.0 (–CH 2 –), 58.9 (–CH 2 –), 50.8 (N–CH 3 ), 43.9 (N–CH 3 ), 43.5 (N–CH 3 ), 24.2 (–CH 3 , AcO), 24.1 (–CH 3 , AcO). HRMS ( m / z ): calculated 1,127.259 and found 1,127.257 ({[Pd- 1b ·(AcO) 2 ](CF 3 SO 3 ) 1 } 1+ ), calculated 489.154 and found 489.153 ({[Pd- 1b ·(AcO) 2 ]} 2+ ). For NMR, IR and ESI-MS analysis of the Pd-1b ·(AcO) 2 (CF 3 SO 3 ) 2 compound, see Supplementary Figs 26–32 . Synthesis of 4·(BArF) 8 molecular cage 10.56 mg of 5,10,15,20-tetrakis(4-carboxyphenyl)porphyrin-Zn II ( 2 , 0.01 mmols) are weighed in a 10 ml flask, then 1 ml of DMF is added. Then, 10 μl of triethylenetriamine dissolved in 0.5 ml of DMF are added to the porphyrin solution. Finally 30 mg of Pd-1b ·(AcO) 2 (CF 3 SO 3 ) 2 (0.02 mmols) complex dissolved in 2.5 ml of DMF are added to the mixture. The solution obtained is heated to 105 °C under reflux for 16 h. After the reaction time, the mixture is cooled to room temperature, filtered through Celite and recrystallized by diethyl ether diffusion. The 4 ·(CF 3 SO 3 ) 8 crystalline solid obtained (extremely low solubility prevented NMR characterization; however, high sensibility of HRMS analysis allowed its mass spectrometry characterization, see Supplementary Fig. 33 ) is suspended in 12 ml of DCM, an excess of NaBArF salt is added (1 to 10 equivalents) and the mixture is stirred vigorously for 16 h. The reaction mixture is filtered. The product is obtained by precipitation with diethyl ether. The purple powder is washed several times with diethyl ether to remove the excess of NaBArF. (Yield: 38.3%). 1 H-NMR (400 MHz, CD 3 CN) δ p.p.m. : 8.60 (dd, 8H, arom-porph), 8.58 (s, 16H, pyrrole ring), 8.35 (dd, J =8 Hz, 8H, arom-porph), 8.30 (d, J =8.5 Hz, 32H, arom-clip), 8.15 (d, J =8.5 Hz, 32H, arom-clip), 8.10 (dd, J =8 Hz, 8H, arom-porph), 7.98 (dd, J =8 Hz, 8H, arom-porph), 7.68 (m, 96H, NaBArF), 4.07 (d, J =13 Hz, 16H, –CH 2 –), 3.70 (m, 16H, –CH 2 –), 3.60 (s, 48H, N–CH 3 ), 3.38 (m, 16H, –CH 2 –), 3.15 (d, J =13 Hz, 16H, –CH 2 –), 2.49 (dd, J =13.5, 16H, –CH 2 –), 2.39 (dd, J =13.5, 16H, –CH 2 –), 1.58 (s, 24H, N–CH 3 ). 13 C-NMR (100 MHz, CD 3 CN) δ p.p.m. : 206.7 (BArF), 166.0 (DMF), 160.4 (BArF), 148.8 (pyrrole ring), 140.4 (arom-clip), 134.6 (BArF), 133.8 (arom-porph), 133.1 (arom-clip), 133.1 (arom-porph), 129.7 (pyrrole ring), 127.1 (arom-clip), 127.1 (arom-porph), 116.6 (BArF), 64.7 (–CH 2 –), 60.2 (–CH 2 –), 59.1 (–CH 2 –), 51.6 (NCH 3 ), 42.6 (NCH 3 ). HRMS ( m / z ): calculated 2,147.893 and found 2,147.893 ({ 4 ·(BArF) 4 } 4+ ); calculated 1,545.701 and found 1,545.702 ({ 4 ·(BArF) 3 } 5+ ), calculated 1,144.239 and found 1,144.242 ({ 4 ·(BArF) 2 } 6+ ); calculated 857.481 and found 857.483 ({ 4 ·(BArF)} 7+ ); calculated 642.413 and found 642.414 ({ 4 ·(BArF)} 8+ ). For NMR and HRMS analysis of the 4 ·(BArF) 8 compound, see Supplementary Figs 34–40 . Preparation and characterization of the fullerene adducts Preparation of C 60 ⊂ 4 ·(BArF) 8 : 2.5 mg of 4· (BArF) 8 nanocapsule (0.2 μmols, 1 equivalent) were dissolved in 100 μl of CH 3 CN. Then one equivalent of C 60 dissolved in 400 μl of toluene was added to the cage solution. The mixture was stirred at room temperature for 5 min. The mixture is filtered and recrystallized by diethyl ether diffusion. 1 H-NMR (400 MHz, CD 3 CN) δ p.p.m. : 8.64 (dd, 8H, arom-porph), 8.55 (s, 16H, pyrrole ring), 8.35 (dd, J =8 Hz, 8H, arom-porph), 8.30 (d, J =8.5 Hz, 32H, arom-clip), 8.14 (d, J =8.5 Hz, 32H, arom-clip), 8.04 (dd, J =8 Hz, 8H, arom-porph), 7.99 (dd, J =8 Hz, 8H, arom-porph), 7.68 (m, 96H, NaBArF), 4.07 (d, J =13 Hz, 16H, –CH 2 –), 3.70 (m, 16H, –CH 2 –), 3.60 (s, 48H, N–CH 3 ), 3.38 (m, 16H, –CH 2 –), 3.15 (d, J =13 Hz, 16H, –CH 2 –), 2.49 (dd, J =13.5, 16H, –CH 2 –), 2.39 (dd, J =13.5, 16H, –CH 2 –), 1.58 (s, 24H, N–CH 3 ). HRMS ( m / z ): calculated 2,328.143 and found 2,328.144 ({C 60 ⊂ 4·( BArF) 4 } 4+ ); calculated 1,689.901 and found 1,689.902 ({C 60 ⊂ 4·( BArF) 3 } 5+ ), calculated 1,264.406 and found 1,264.408 ({C 60 ⊂ 4·( BArF) 2 } 6+ ); calculated 960.339 and found 960.341 ({C 60 ⊂ 4·( BArF)} 7+ ); calculated 732.413 and found 732.415 ({C 60 ⊂ 4·( BArF)} 8+ ). Preparation of C 70 ⊂ 4 ·(BArF) 8 : 2.5 mg of 4· (BArF) 8 nanocapsule (0.2 μmols, one equivalent) was dissolved in 100 μl of CH 3 CN. Then one equivalent of C 70 dissolved in 400 μl of toluene was added to the cage solution. The mixture was stirred at room temperature for 5 min. The mixture is filtered and recrystallized by diethyl ether diffusion. 1 H-NMR (400 MHz, CD 3 CN) δ p.p.m. : 8.66 (dd, J =8 Hz, 8H, arom-porph), 8.48 (s, 16H, pyrrole ring), 8.33 (dd, 8H, arom-porph), 8.33 (d, J=8.5 Hz, 32H, arom-clip), 8.18 (d, J =8.5 Hz, 32H, arom-clip), 8.00 (m, J =8 Hz, 8H, arom-porph), 7.97 (m, J =8 Hz, 8H, arom-porph), 7.68 (m, 137H, NaBArF), 4.09 (d, J =13 Hz, 16H, –CH 2 –), 3.70 (m, 16H, –CH 2 –), 3.60 (s, 48H, N–CH 3 ), 3.38 (m, 16H, –CH 2 –), 3.15 (d, J =13 Hz, 16H, –CH 2 –), 2.49 (dd, J =13.5, 16H, –CH 2 –), 2.39 (dd, J =13.5, 16H, –CH 2 –), 1.59 (s, 24H, N–CH 3 ). HRMS ( m / z ): calculated 2,358.143 and found 2,358.141 ({C 70 ⊂ 4· (BArF) 4 } 4+ ); calculated 1,713.901 and found 1,713.900 ({C 70 ⊂ 4· (BArF) 3 } 5+ ), calculated 1,284.406 and found 1,284.409 ({C 70 ⊂ 4· (BArF) 2 } 6+ ); calculated 977.624 and found 977.625 ({C 70 ⊂ 4· (BArF)} 7+ ); calculated 747.413 and found 747.413 ({C 70 ⊂ 4· (BArF)} 8+ ). Preparation of [C 60 ]PCBM ⊂ 4 ·(BArF) 8 : 2.5 mg of 4· (BArF) 8 nanocapsule (0.2 μmols, one equivalent) were dissolved in 100 μl of CH 3 CN. Then one equivalent of [C 60 ]PCBM dissolved in 400 μl of toluene was added to the cage solution. The mixture was stirred at room temperature for 5 min. The mixture is filtered and recrystallized by diethyl ether diffusion. 1 H-NMR (400 MHz, CD 3 CN) δ p.p.m. : 8.60 (dd, J =8.0 Hz, 8H, arom-porph), 8.50 (s, 16H, pyrrole ring), 8.35 (dd, J =8.0 Hz, 8H, arom-porph), 8.32 (d, J =8.5 Hz, 32H, arom-clip), 8.13 (d, J =8.5 Hz, 32H, arom-clip), 7.99 (m, J =8 Hz, 8H, arom-porph), 7.92 (m, J =8 Hz, 8H, arom-porph), 142 (m, 96H, NaBArF), 4.09 (d, J =13 Hz, 16H, –CH 2 –), 3.67 (m, 16H, –CH 2 –), 3.60 (s, 48H, N–CH 3 ), 3.38 (m, 16H, –CH 2 –), 3.15 (d, J =13 Hz, 16H, –CH 2 –), 2.49 (dd, J =13.5, 16H, –CH 2 –), 2.40 (dd, J =13.5, 16H, –CH 2 –), 1.59 (s, 24H, N–CH 3 ). HRMS ( m / z ): calculated 2,375.668 and found 2,375.667 ({[C 60 ]PCBM ⊂ 4· (BArF) 4 } 4+ ); calculated 1,727.921 and found 1,727.923 ({[C 60 ]PCBM ⊂ 4· (BArF) 3 } 5+ ), calculated 1,296.089 and found 1,296.088 ({[C 60 ]PCBM ⊂ 4· (BArF) 2 } 6+ ); calculated 987.639 and found 987.636 ({[C 60 ]PCBM ⊂ 4· (BArF)} 7+ ); calculated 756.175 and found 756.173 ({[C 60 ]PCBM ⊂ 4· (BArF)} 8+ ). For NMR and HRMS analysis of the host–guest adducts, see Supplementary Figs 41–55 . General procedures for UV–vis and fluorescence titrations Host–guest interactions in solution were studied by UV–vis and fluorescence spectroscopy. The UV–vis titration experiments between 4 ·(BArF) 8 (4.32 × 10 −7 M) and the different fullerenes tested (1.39 × 10 −5 M) were performed by using toluene/acetonitrile (9/1) as solvent. The cage concentration was kept constant. The C 60 (3.46 × 10 −6 M) titration was repeated using a constant concentration of 4 ·(BArF) 8 of 1.08 × 10 −7 M. A magnetic stir bar and 2 ml of nanocapsule solution were added to the cuvette, then it was inserted into the spectrometer and the stirrer activated and the substrate added. The stoichiometry of the complexes was studied using the method of continuous variations. Solutions of nanocapsule 4 ·(BArF) 8 and fullerenes (4.32 × 10 −7 M) in toluene/acetonitrile (9/1) were mixed at different ratios. All the experiments were carried out at 22 °C. The fluorescence titration for C 60 was performed under the same conditions of the UV–vis titration. C 70 fluorescence titration experiment was performed using a 1.08 × 10 −8 M solution of 4 ·(BArF) 8 and 3.46 × 10 −7 M solution of C 70 . A 9/1 mixture of toluene/acetonitrile was used as solvent and the cage concentration was kept constant. The data obtained from the UV–vis and the fluorescence spectrophotometric titrations were analysed using the software Origin Pro 8 and SPECFIT 3.0 from Spectrum Software Associates, Marlborough, MA, U.S.A. (SpecSoft@compuserve.com), which uses a global system with expanded factor analysis and Marquardt least-squares minimization to obtain globally optimized parameters. For UV–vis titrations of the host–guest adducts, see Supplementary Figs 56–60 . Diffusion-ordered NMR spectroscopy experiments Diffusion-ordered NMR experiments (DOSY NMR) of Pd-1b ·(AcO) 2 (CF 3 SO 3 ) 2 , 4 ·(BArF) 8 , C 60 ⊂ 4 ·(BArF) 8 and C 70 ⊂ 4 ·(BArF) 8 , allow the determination of the translational self-diffusion coefficients ( D ) for these species in acetonitrile solution. Making use of the Stokes–Einstein equation (equation 1), the hydrodynamic radii ( r H ) for the diffused species can be calculated from the D value (see obtained values on Supplementary Table 1). where k is the Boltzmann constant, T is the temperature, and η is the viscosity of the solvent ( η (CH 3 CN)=0.35 mPa s) (ref. 56 ). The DOSY spectra were acquired using the LEDBP pulse sequence using 16 transients and eight dummy scans, at 298 K. The diffusion time D was 150 ms and the total diffusion-encoding gradient duration ( d ) was 1.1 ms. Sixteen values of diffusion-encoding gradient were used, varying from approximately 1 to 50 G cm −1 in equal steps of gradient squared. Data were acquired and processed using the automated ‘dosy’ and ‘dosy2d’ macros incorporated into the TOPSPIN v2.1 software package (Bruker Biospin, Rheinstetten, Germany). For DOSY-NMR experiments of the host–guest adducts, see Supplementary Figs 61–64 . X-ray diffraction studies details Crystallographic data for Pd-1b ·(AcO) 2 (CF 3 SO 3 ) 2 were collected using Bruker-AXS SMART-APEXII CCD diffractometer (MoK α , λ =0.71073 Å). Indexing was performed using APEX2 (Difference Vectors method). Data integration and reduction were performed using SaintPlus 6.01. Absorption correction was performed by multi-scan method implemented in SADABS. The structure was solved using SHELXS-97 and refined using SHELXL-97 contained in SHELXTL program. All hydrogen atoms were placed using a riding model. Their positions were constrained relative to their parent atom using the appropriate HFIX command in SHELXL-97. See Supplementary Data 2 . Crystallographic data for 4 ·(BArF) 8 , C 60 ⊂ 4 ·(BArF) 8 and C 70 ⊂ 4 ·(BArF) 8 samples were collected at the XALOC beamline of the ALBA synchrotron at 100 K using a MD2M single-axis diffractometer (Maatel, France) and a Pilatus 6 M detector (Dectris, Switzerland). Due to their sensitivity to solvent loss, crystals of the three complexes were mounted in thin glass capillaries and cryopreserved at 100 K. Single crystals were introduced into the capillary suspended in a small volume of ether/DMF (solution used to grow the crystal saturated with ether). The data sets were collected on omega single-axis scans with 1-s per frame exposures at λ =0.82656 Å. The crystals were diffracting at a moderate resolution (2.3 Å) (see Supplementary Fig. 67 ) and showed degradation due to radiation damage, as seen from the intensities and resolution of the reflections after 266 (for 4 ·(BArF) 8 ; see Supplementary Fig. 67 ), 220 (for C 60 ⊂ 4 ·(BArF) 8 ; see Supplementary Fig. 67 ) and 178 (C 70 ⊂ 4 ·(BArF) 8 ; see Supplementary Fig. 67 ) images. This poor density and fast degradation is attributed to the high symmetry, solvent loss and severe motions of the solvents (volatile ether) and counteranion molecules (BArF) in the large cavities of the crystal lattice. The three structures were solved by charge flipping method using the code Superflip [57] and refined by the full matrix least-squares based of F 2 using SHELX97 (ref. 58 ). Although the limited quality of the data ( Supplementary Table 5 ) did not allow locating the counteranions and solvent molecules in the unit cell, the atomic positions of the atoms composing the cage and disordered C 60 and C 70 could be determined. For the same reasons, the atoms have been refined only isotropically. We provide, as additional data sets, preliminary CIF files extracted from partial refinement X-ray diffraction data, see Supplementary Data 3–5 . For X-ray diffraction data of 4 ·(BArF) 8, C 60 ⊂ 4 ·(BArF) 8 and C 70 ⊂ 4 ·(BArF) 8 , see Supplementary Figs 65–69 . Computational details All DFT calculations were performed using the ADF 2010 program. The molecular orbitals were expanded in an uncontracted set of Slater-type orbitals of double-ζ (DZ), and double-ζ (DZP) and triple-ζ (TZP) quality that contained diffuse functions and one set of polarization functions. The Frozen core approximation was used along the self-consistent field procedure. Scalar relativistic corrections have been included self consistently by using the zeroth order approximation. Energies and gradients were calculated by using the local density approximation (Slater exchange) with non-local corrections for exchange (Becke88) and correlation (Lee–Yang–Parr) included self consistently (that is, BLYP functional). Solvent effects (acetonitrile) were included through the use of COSMO approach. All structures were optimized using the QUILD program, which functions as a wrapper around the ADF program. QUILD uses improved geometry-optimization techniques, such as adapted delocalized coordinates and specially constructed model Hessians. When necessary, Cl − counteranions have been used instead of BArF − for reducing computational complexity. See the Supplementary Discussion 1 for a detailed description and corresponding references. For DFT structures of 4 ·(BArF) 8 and its host–guest adducts, see Supplementary Figs 70–72 and Supplementary Data 1 . How to cite this article: García-Simón, C. et al . Sponge-like molecular cage for purification of fullerenes. Nat. Commun. 5:5557 doi: 10.1038/ncomms6557 (2014).